Broadband high photoresponse from pure monolayer graphene photodetector Graphene has attracted large interest in photonic applications owing to its promising optical properties, especially its ability to absorb light over a broad wavelength range, which has lead to several studies on pure monolayer graphene-based photodetectors. However, the maximum responsivity of these photodetectors is below 10 mA W −1 , which significantly limits their potential for applications. Here we report high photoresponsivity (with high photoconductive gain) of 8.61 A W −1 in pure monolayer graphene photodetectors, about three orders of magnitude higher than those reported in the literature, by introducing electron trapping centres and by creating a bandgap in graphene through band structure engineering. In addition, broadband photoresponse with high photoresponsivity from the visible to the mid-infrared is experimentally demonstrated. To the best of our knowledge, this work demonstrates the broadest photoresponse with high photoresponsivity from pure monolayer graphene photodetectors, proving the potential of graphene as a promising material for efficient optoelectronic devices. Graphene, a two dimensional allotrope of carbon atoms on a honeycomb lattice with unique band structure, has recently attracted significant interest in photonic applications for realizing, for example, transparent electrodes [1] , optical modulator [2] , polarizer [3] , surface plasmonic devices [4] , [5] and photodetectors [6] , [7] , [8] , [9] . One of the most impressive advantages is its ability to absorb ~2.3% of incident light over a broad wavelength range despite its one-atom layer thickness [10] . This advantage makes the realization of broadband photodetectors possible, far exceeding the bandwidth of the current photodetectors. In addition, graphene also shows high mobility, which is promising for applications in ultrafast detection. Based on these properties, several works have been reported on the realization of graphene-based photodetectors in a field-effect transistor (FET) structure [6] , [7] , [8] , [9] . However, the highest photoresponsivity (photo-generated current per incident optical power) is <10 mAW −1 . Although some strategies such as using surface plasmons [11] , [12] or microcavity [13] have been adopted to enhance the performance of the graphene photodetector, the photoresponsivity is still as low as several tens of mAW −1 and the fabrication processes are complex. In conventional FET-based graphene photodetectors, the low photoresponsivity is mainly attributed to the low optical absorption in monolayer graphene and the short recombination lifetime (on the scale of a picosecond) of the photo-generated carriers, leading to a low internal quantum efficiency of ~6–16% ( [6] ). Thus, to achieve high photoresponsivity, one should increase either the absorption efficiency of graphene [11] , [12] , [13] or the lifetime of the photo-excited carriers, while still maintaining the high mobility by modifying the properties of graphene. In addition, although pure monolayer graphene photodetectors have been predicted as having ultra-wideband operation in theory [10] , all of the reported results based on pure monolayer graphene photodetectors are realized in the visible or the near-infrared ranges [6] , [7] , [8] , [9] , [11] , [12] , [13] , [14] , [15] and not demonstrated in the longer wavelength range. Band structure engineering of graphene has been widely investigated. A bandgap can be created in graphene for electronic applications, for example, by patterning graphene nanoribbon or nanomesh structures through electron-beam lithography [16] , nanowire shadow mask etching [17] , block copolymer lithography [18] and/or unzipping of carbon nanotubes [19] , [20] . On the other hand, various defect states can also be created in graphene by defect engineering [21] for manipulating electrical [22] , [23] , chemical [23] , [24] and magnetic [25] , [26] properties. Here we introduce defect midgap states band (MGB) [27] , as well as a bandgap in graphene through a Titanium (Ti) sacrificial layer fabrication method for achieving high photoresponse. Through this scheme, we have demonstrated a high photoresponsivity of 8.61 AW −1 , which are about three orders of magnitude higher than those in previous reports from pure monolayer graphene photodetectors. The methodology presented here can provide a new avenue for the development of graphene-based broadband high performance photodetectors and other optoelectronic devices. In addition to a high photoresponsivity, we have demonstrated the broadest photoresponse from the visible (532 nm) up to the mid-infrared (~10 μm) in a single pure graphene photodetector. We noted that graphene hybrid photodetector with an ultrahigh photoconductive gain has been recently demonstrated where semiconductor quantum dots were adopted as light absorbers and graphene was used as an ultrafast transport medium [28] . While, as the photoresponse of these devices are dependent on the properties of the quantum dots, the broadband advantage of the graphene is lost, for example, the hybrid graphene photodetector does not work in the important mid-infrared regime. Compared with the traditional mid-infrared photodetectors such as HgCdTe (HCT) and quantum well infrared photodetector, the proposed graphene photodetector possesses the advantages of a lower cost and a lower operation power, and it is compatible with the complementary metal-oxide-semiconductor technologies, while still maintaining a high photoresponse. Concept of the proposed graphene photodetector To increase the photoresponsivity of pure graphene photodetectors, apart from the prevailing methods of increasing the absorption efficiency of graphene [11] , [12] , [13] , one could also increase the lifetime of the photo-generated electrons. However, owing to the fast interband and intraband recombination rate of a few picoseconds of the photo-generated electrons [29] ( Fig. 1a ), even though a carrier multiexcitation generation (MEG) process has been theoretically predicted [30] in a perfect graphene with a multiplication factor of approximately four by the impact ionization process (also called the inverse Auger recombination (AR)), up to now no multiplication effect has been experimentally observed in pure graphene sheet (we noticed that the MEG effect in graphene was observed experimentally and reported almost simultaneously [31] at the time of this publication, confirming the high efficiency of carrier-carrier scattering in graphene.). 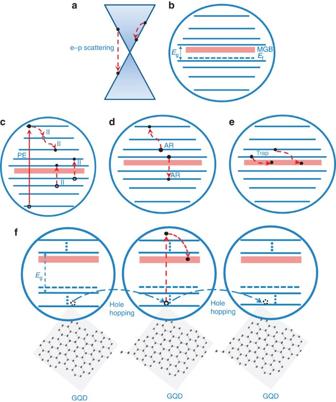Figure 1: Energy band diagram and concept of the graphene photodetector. (a) Band structure diagram of pure graphene sheet. The red arrows indicate the intraband and interband electron–phonon scattering. (b) Energy band diagram of the GQD including the MGB.Egis the quantum-confined bandgap. Shadow region indicates the MGB, andEfis the Fermi energy level. (c) Generation of an electron-hole pair via photon excitation (PE) followed by the impact ionization (II) process. When the electron is excited into much higher energy of the conduction band, the II cascade of carriers occurs. Each cascade step involves electron-hole pair generation. Owing to the high efficiency of the carrier-carrier scattering in graphene, MEG effect exists. It is noted that holes can also contribute to the carrier MEG process assisted by an external electrical field, to be explained in the latter part of the paper. (d) Excitation of an electron to a higher-energy level in the conduction band via the AR process, followed by recombination of another electron with a hole in the valence band. (e) Trapping/relaxation process of the excited electrons to the MGB. (f) Graphene photoconductive channel consists of GQD arrays. The photo-excited and the secondary electrons are captured by the MGB having a long lifetime. Before the trapped electrons are recombined, the corresponding holes can circulate many times in the photoconductive channel, thus achieving a high photoconductive gain. Figure 1: Energy band diagram and concept of the graphene photodetector. ( a ) Band structure diagram of pure graphene sheet. The red arrows indicate the intraband and interband electron–phonon scattering. ( b ) Energy band diagram of the GQD including the MGB. E g is the quantum-confined bandgap. Shadow region indicates the MGB, and E f is the Fermi energy level. ( c ) Generation of an electron-hole pair via photon excitation (PE) followed by the impact ionization (II) process. When the electron is excited into much higher energy of the conduction band, the II cascade of carriers occurs. Each cascade step involves electron-hole pair generation. Owing to the high efficiency of the carrier-carrier scattering in graphene, MEG effect exists. It is noted that holes can also contribute to the carrier MEG process assisted by an external electrical field, to be explained in the latter part of the paper. ( d ) Excitation of an electron to a higher-energy level in the conduction band via the AR process, followed by recombination of another electron with a hole in the valence band. ( e ) Trapping/relaxation process of the excited electrons to the MGB. ( f ) Graphene photoconductive channel consists of GQD arrays. The photo-excited and the secondary electrons are captured by the MGB having a long lifetime. Before the trapped electrons are recombined, the corresponding holes can circulate many times in the photoconductive channel, thus achieving a high photoconductive gain. Full size image The detailed physical picture on how a high photoconductive gain is achieved in this work is depicted as follows: we first process the graphene sheet into a graphene quantum dot-like (GQD)-arrays structure; then defect MGB electron trapping centres are formed on the boundary and surface of the GQDs and a bandgap is created due to the quantum confinement. The corresponding energy band diagram is shown in Fig. 1b . The sequence of the carrier MEG and trapping in the MGB is depicted in Fig. 1c–e . As shown in Fig. 1c , the impact ionization (II) process exists in the GQDs: one photo-excited electron relaxes to a lower-energy state within the conduction band, exciting a valence band electron into the conduction band. Meanwhile, electrons of the conduction band will be involved in the AR process ( Fig. 1d ): an electron is scattered from the conduction band into the valence band, while simultaneously the released energy is transferred to another electron, which is excited to a higher-energy state in the conduction band. Despite the competing processes between II and AR, II can be more efficient than the AR process in quantum-confined systems [32] because of the asymmetry between the II and AR [33] . Therefore, carrier multiplication (the MEG effect) occurs, which generates more secondary electrons in the conduction band, see Fig. 1c , thus enhancing the electron generation efficiency. As a bandgap is formed, the electron–phonon scattering rate from the conduction band to valence band decreases [34] so that more photo-generated, as well as the secondary-generated electrons can be trapped in the MGB ( Fig. 1e ). It is noted that holes can also contribute to the carrier MEG process assisted by an external electrical field, as illustrated in the latter part of the paper. When the photo-generated and the secondary-generated electrons are trapped in the MGB, the related holes can be recirculated many times through hopping within the lifetime of the MGB trapped electrons ( Fig. 1f ); thus a photoconductive gain is achieved. Owing to the relatively long electron trapping time in the MGB together with the high efficiency of the carrier MEG effect in graphene, we expect a high photoresponse can be achieved in GQD array photodetectors. Device fabrication and characterization We fabricated pure graphene photodetectors in a FET structure through a Ti etching fabrication method, which is shown schematically in Fig. 2a–d and discussed in more details in Methods. Three devices were fabricated and compared: Sample A is based on a pristine graphene structure (without the Ti layer fabrication); Sample B is a GQD arrays structure fabricated with a ~2-nm thick Ti layer; and Sample C is a GQD arrays structure fabricated with a ~20-nm thick Ti layer. Raman spectra measurements were used to characterize the density of defects of these samples [35] (see Methods). As shown in Fig. 3a , a higher number of defects were observed in Sample C than in Sample B due to the higher Raman I D / I G ratio [36] , [37] ( I D and I G are the D-band and G-band Raman intensities, respectively). For Sample C, the average crystallite size of the GQDs L a is estimated to be ~7.5 nm from [38] L a ( nm )=(2.4 × 10 −10 )λ( nm ) 4 ( I D / I G ) −1 , where λ=532 nm is the wavelength of the Raman signal. Similarly, Sample B has an average GQD size of ~20.5 nm. The electrical characteristics of the Samples A and C are shown in Fig. 3b , respectively. 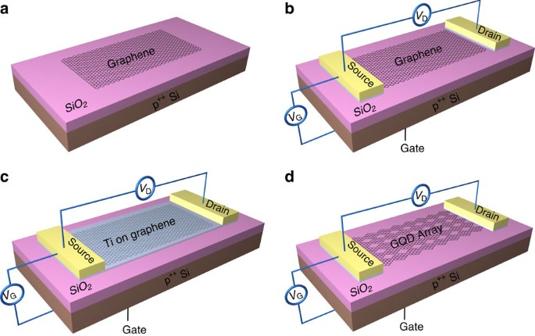Figure 2: Fabrication process of the device. (a) A monolayer graphene was mechanically exfoliated onto a 285 nm SiO2/Si substrate. (b) The graphene photodetector was processed into a FET structure. Two electrodes (that is, the source and the drain terminals) of Ti/Au (20 nm/80 nm) were fabricated on the graphene by photolithography and lift-off processes. The gate terminal was fabricated on the bottom of the Si substrate. (c) A thin nm-scale Ti sacrificial layer was deposited onto the graphene by electron-beam evaporation. (d) The Ti sacrificial layer was removed via wet etching, and then GQD array structure with various quantum dot (QD) sizes can be formed on the Si substrate depending on the thickness of the Ti layer. For Sample A, the transfer curve shows an ambipolar transfer property with the Dirac point at ~60 V, while it is at ~80 V for Sample C. Figure 2: Fabrication process of the device. ( a ) A monolayer graphene was mechanically exfoliated onto a 285 nm SiO 2 /Si substrate. ( b ) The graphene photodetector was processed into a FET structure. Two electrodes (that is, the source and the drain terminals) of Ti/Au (20 nm/80 nm) were fabricated on the graphene by photolithography and lift-off processes. The gate terminal was fabricated on the bottom of the Si substrate. ( c ) A thin nm-scale Ti sacrificial layer was deposited onto the graphene by electron-beam evaporation. ( d ) The Ti sacrificial layer was removed via wet etching, and then GQD array structure with various quantum dot (QD) sizes can be formed on the Si substrate depending on the thickness of the Ti layer. 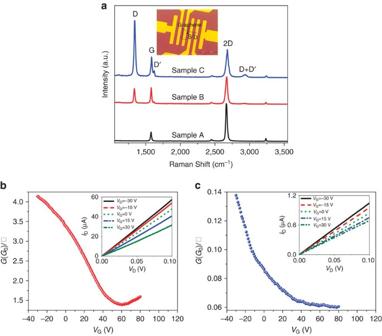Figure 3: Raman spectra and electrical characteristics. (a) Raman spectra of the pristine graphene (Sample A, black curve) and the processed graphene samples fabricated with a 2-nm thick Ti layer (Sample B, red curve) and a 20-nm thick Ti layer (Sample C, blue curve). The Raman spectra were excited at 532 nm with an incident power <1 mW (laser spot diameter of 500 nm). The results show that almost no defect states are in Sample A as only G-band (1,578 cm−1) and 2D band (2,666 cm−1) are observed, while Sample C has the largest number of defect states as the ratio of the D-band (1,338 cm−1) to the G-band (1,578 cm−1) Raman intensities is the highest. The inset shows the microscope image of Sample C, where the size (~20 μm × 10 μm) of the monolayer graphene and the source (represented by S) and the drain (represented by D) terminals are indicated. (b) The electrical characteristics as a function of the gate voltage (transfer curve) of Sample A; the inset shows the current–voltage (I–V) curves of this sample under different gate voltages. The Dirac point occurs atVG~60V. (c) The electrical characteristics as a function of the gate voltage of Sample C; the inset shows theI–Vcurves of this sample under different gate voltages. Full size image Figure 3: Raman spectra and electrical characteristics. ( a ) Raman spectra of the pristine graphene (Sample A, black curve) and the processed graphene samples fabricated with a 2-nm thick Ti layer (Sample B, red curve) and a 20-nm thick Ti layer (Sample C, blue curve). The Raman spectra were excited at 532 nm with an incident power <1 mW (laser spot diameter of 500 nm). The results show that almost no defect states are in Sample A as only G-band (1,578 cm −1 ) and 2D band (2,666 cm −1 ) are observed, while Sample C has the largest number of defect states as the ratio of the D-band (1,338 cm −1 ) to the G-band (1,578 cm −1 ) Raman intensities is the highest. The inset shows the microscope image of Sample C, where the size (~20 μm × 10 μm) of the monolayer graphene and the source (represented by S) and the drain (represented by D) terminals are indicated. ( b ) The electrical characteristics as a function of the gate voltage (transfer curve) of Sample A; the inset shows the current–voltage ( I – V ) curves of this sample under different gate voltages. The Dirac point occurs at V G ~60V. ( c ) The electrical characteristics as a function of the gate voltage of Sample C; the inset shows the I – V curves of this sample under different gate voltages. Full size image Carrier transport in the processed graphene device To investigate the carrier transport properties of the processed graphene device, i.e. the GQD arrays device (refer to Sample C in the latter part of the paper, if not specified), we measured the electrical properties of the device at different temperatures ( Fig. 4a–c ). The observations indicate the carrier transport in the graphene FET photodetector is influenced by the Coulomb blockade of charges [39] (see Methods). Figure. 4b shows the current ( I ) versus temperature ( T ) characteristics in the temperature range 8–290 K, that is, the temperature dependence of the conductivity. The best fit of the temperature-dependent data is obtained with the T −1/3 curve fitting (inset, Fig. 4b ), but not with the T −1 or T −1/2 fitting (see Supplementary Fig. S1 and Supplementary Note 1 ). These results show that variable range hopping (VRH), frequently observed in disordered systems including carbon-related materials [40] , is the main carrier transport mechanism (see Methods), which involves consecutive hopping process between two localized states. It is thus confirmed that the processed device is formed by GQD arrays with polydispersed GQDs. 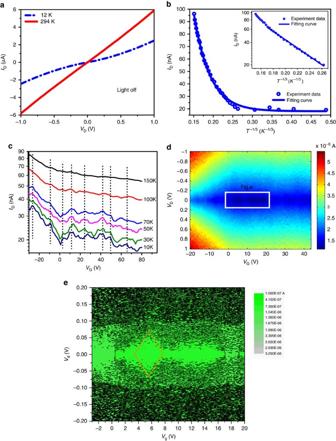Figure 4: Carrier transport in the proposed graphene photodetector. (a) TheI–Vcharacteristics of Sample C at 294 K and 12 K, respectively. The fact that theI–Vcharacteristic is linear at 294 K, while becomes nonlinear and maintains highly symmetric indicates that a carrier transport barrier is formed in the GQD array structure, which is caused by the Coulomb blockade of charges. (b) The temperature dependence of the drain current of Sample C is best fitted in aT−1/3scale. The results show that VRH is the main carrier transport mechanism. The inset shows a good liner fitting of the photocurrent in the logarithmic scale with respect toT−1/3. This suggests that the processed graphene device consists of polydispersed GQDs. (c) The transfer curves of Sample C at different temperatures, in which strong temperature dependence is shown. (d) Differential conductance as a function ofVGandVDof Sample C at 12 K and (e) its magnification plot. The diamond-shaped region suggests the Coulomb blockade effect influences the carrier transport. Figure 4: Carrier transport in the proposed graphene photodetector. ( a ) The I – V characteristics of Sample C at 294 K and 12 K, respectively. The fact that the I – V characteristic is linear at 294 K, while becomes nonlinear and maintains highly symmetric indicates that a carrier transport barrier is formed in the GQD array structure, which is caused by the Coulomb blockade of charges. ( b ) The temperature dependence of the drain current of Sample C is best fitted in a T −1/3 scale. The results show that VRH is the main carrier transport mechanism. The inset shows a good liner fitting of the photocurrent in the logarithmic scale with respect to T −1/3 . This suggests that the processed graphene device consists of polydispersed GQDs. ( c ) The transfer curves of Sample C at different temperatures, in which strong temperature dependence is shown. ( d ) Differential conductance as a function of V G and V D of Sample C at 12 K and ( e ) its magnification plot. The diamond-shaped region suggests the Coulomb blockade effect influences the carrier transport. Full size image To further study the Coulomb blockade effect in the processed graphene device, the temperature-dependent transfer curves are also measured ( Fig. 4c ). Obvious oscillations appear in the transfer curves at low temperatures and these oscillation peaks are gradually broadened with the temperature and disappear when the temperature is higher than 150 K. These observations are clear evidence of the Coulomb blockade effect [41] , [42] . To calculate the charge energy of the GQDs, we measured differential conductance (d I /d V ) as functions of V G and V D , as shown in Fig. 4d . By calculating the height of the diamond-shape regions [16] , [39] , we obtain an energy gap of about 75 meV, consistent with the estimated value of ~88 meV calculated from , where ν F ≈ 10 6 ms −1 is the Fermi velocity in graphene, and W is the average size of the GQDs (~7.5 nm). Broadband photoresponse measurement We measured the photoresponse characteristics of the processed graphene device at 20-mV source-drain bias and zero gate voltage, with illuminations on the whole device at various wavelengths, and at low temperatures (see Fig. 5 ). Light sources at the visible (532 nm), the near-infrared (1.47 μm) and the mid-infrared (9.9 μm, 10.1 μm and 10.31 μm) were used in the photoresponse measurements. For comparison, the photoresponse of the pristine graphene device was also measured (see Supplementary Fig. S2 and Supplementary Note 2 ) and no obvious response was observed at a low optical input power density ~633 mWcm −2 , which agrees with the previous results (only a low responsivity of about 10 mAW −1 was reported under a high optical pumping of 10 8 mW cm −2 ). The photoresponse of the processed graphene device is shown in Fig. 5a–f , respectively, for the visible, the near-infrared and the mid-infrared illuminations. The processed graphene device shows high photoresponse in the whole tested wavelength range (high photoresponsivity of 1.25 AW −1 , 0.2 AW −1 and 0.4 AW −1 in the visible, near-infrared and mid-infrared ranges, respectively). These values are about two-three orders higher than those reported in the literature based on pure monolayer graphene photodetectors. More importantly, to the best of our knowledge, this is the broadest range reported for a single graphene-based photodetector device. 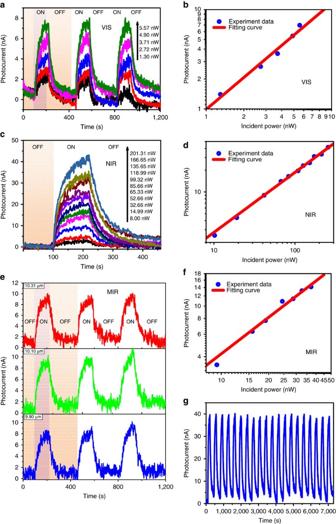Figure 5: Broadband photoresponse measurements of the graphene photodetector. (a) Time-dependent photocurrent measurements of Sample C when optically pumped in (a) the visible (VIS) (532 nm), (c) the near-infrared (NIR) (1.47 μm) and (e) the mid-infrared (MIR) (~10 μm) ranges. The GQD photodetector shows high photoresponses: ~1.25 AW−1, 0.2 AW−1and 0.4 AW−1in the visible, NIR and MIR ranges, respectively.b,dand f show the power dependence of the photocurrents in the three ranges, respectively, where both axes are in the logarithmic scale. The results also demonstrate that the proposed graphene photodetector also possesses a high photosensitivity property, capable of a nW-level input optical power detection. (g) The time-dependent photocurrent measurement over a 20-periods on–off operation under a NIR light (1.47 μm) illumination, demonstrating the reliability of the photodetector. Figure 5: Broadband photoresponse measurements of the graphene photodetector. ( a ) Time-dependent photocurrent measurements of Sample C when optically pumped in ( a ) the visible (VIS) (532 nm), ( c ) the near-infrared (NIR) (1.47 μm) and ( e ) the mid-infrared (MIR) (~10 μm) ranges. The GQD photodetector shows high photoresponses: ~1.25 AW −1 , 0.2 AW −1 and 0.4 AW −1 in the visible, NIR and MIR ranges, respectively. b , d and f show the power dependence of the photocurrents in the three ranges, respectively, where both axes are in the logarithmic scale. The results also demonstrate that the proposed graphene photodetector also possesses a high photosensitivity property, capable of a nW-level input optical power detection. ( g ) The time-dependent photocurrent measurement over a 20-periods on–off operation under a NIR light (1.47 μm) illumination, demonstrating the reliability of the photodetector. Full size image The proposed graphene photodetector also possesses high sensitivity capable of nW-level optical power detection, demonstrated in Fig. 5b . The power dependence of the photodetector is also shown at different wavelength illuminations ( Fig. 5b ). The photoresponse can be expressed by a power law I pc ∝ P γ , where I pc is the photocurrent and P is the power of the illumination. For the visible, near-infrared and mid-infrared illuminations, γ is 1.07, 0.83 and 0.95, respectively. The non-unity exponentials are the result of complex processes of electron-hole generation, trapping and recombination [43] , implying complex MGB electron trapping and carrier transport in the processed graphene photodetector. Dependence on temperature and voltage and GQDs size The bias dependence of the photoresponse of Sample C is shown in Fig. 6a . As the bias increases from zero to 0.1 V, the photoresponsivity increases up to 8.61 A W −1 correspondingly. The temperature-dependent characteristics of Sample C are shown in Fig. 6b . The results show a strong dependence of the temperature on the photoresponse of the detector. The decrease of the photoresponse with the temperature could be understood as: with the increase of temperature a faster recombination of captured electrons in the MGB states occurs, thus the photoresponse is reduced. 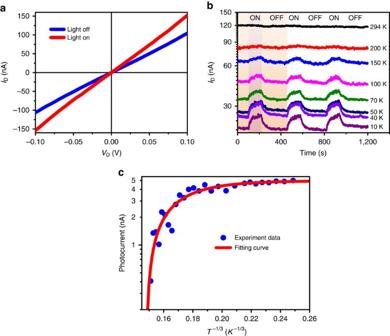Figure 6: Temperature and time dependence of the photocurrent. (a) theI–Vcurves of Sample C with and without 532 nm illuminations. A high photoresponsivity of 8.61 AW-1is achieved at aVDvoltage of 0.1 V. (b) Time-dependent photocurrent measurements at different temperatures under the visible light illumination. (c) Temperature dependence of the photocurrent of Sample C. The photoresponse decreases with the temperature, shown inbandc, resulting from a faster recombination of captured electrons in the MGB at a higher temperature, thus the lifetime of these trapped electrons is reduced. Figure 6: Temperature and time dependence of the photocurrent. ( a ) the I – V curves of Sample C with and without 532 nm illuminations. A high photoresponsivity of 8.61 AW -1 is achieved at a V D voltage of 0.1 V. ( b ) Time-dependent photocurrent measurements at different temperatures under the visible light illumination. ( c ) Temperature dependence of the photocurrent of Sample C. The photoresponse decreases with the temperature, shown in b and c , resulting from a faster recombination of captured electrons in the MGB at a higher temperature, thus the lifetime of these trapped electrons is reduced. Full size image The gate-bias dependence of photoresponse of Sample C is shown in Fig. 7a . As the gate-bias decreases from +20 V to −20 V, the photocurrent increases and the device becomes a more p -type material seen from the transport characteristics in Fig. 3c . This is in contrary to the normal understanding that the electron-hole pair generation by direct photoexcitation would be decreased as the quasi-Fermi level moves below the valence band edge (fewer valence band states are filled with electrons). The observed gate-bias dependence of the photocurrent, we believe, is attributed to the effective electron-hole pair generations by the hole impact ionization assisted by the external electrical field, which was also observed in the carbon nanotube system [44] . As shown in Fig. 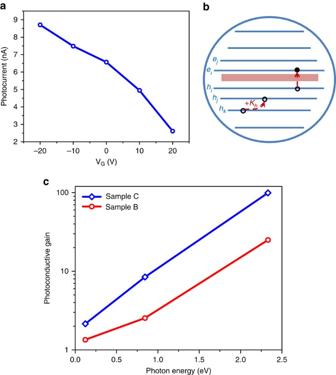Figure 7: Photoresponse dependence on the gate voltage and photon energy, and GQD sizes. (a) The gate voltage dependence of the photoresponse characteristics of Sample C. The increase of the photocurrent with a decrease of the gate voltage can be attributed to the hole impact ionization effect assisted by the external electrical field. As the gate-bias decreases (the quasi-Fermi level decreases, seeFig. 3c), more holes are involved in the impact ionization process to generate more electron-hole pairs. Thus, there is a competing effect between the hole impact ionization and the direct photoexcitation. The former is more efficient than the latter when the material is converted to be morep-type. (b) Hole impact ionization process in the processed graphene photodetector. The rest mass energy of the hole in the high energy levelhkis combined with the kinetic energyKhto create a lower-energy hole and electron-hole pairs as:hk+Kh→hj+n× (e+h) whereKhis the kinetic energy of holes induced by the external electric field.hkandhjindicate the higher-energy and the lower-energy level holes, respectively, (e+h) refer to electron-hole pairs andnis an integer. Thus, with an external electrical field, more electron-hole pairs can be generated through hole impact ionization. (c) The photoconductive gain spectra of Sample B and Sample C, respectively, at different photon excitation energies. The photoconductive gain rises as the photon energy increases, which can be attributed to the increase of the carrier MEG effect. With a higher photon energy excitation (532 nm), a photo-generated electron occupies a higher-energy level and generates multiple secondary electrons when scattering to the lower-energy levels in the conduction band through the MEG process, thus leading to a larger number of the captured electrons in the defect MGB. 7b , the rest mass energy of one photo-excited hole in a higher-energy level is combined with the kinetic energy to create a lower-energy hole plus several electron-hole pairs, expressed as: Figure 7: Photoresponse dependence on the gate voltage and photon energy, and GQD sizes. ( a ) The gate voltage dependence of the photoresponse characteristics of Sample C. The increase of the photocurrent with a decrease of the gate voltage can be attributed to the hole impact ionization effect assisted by the external electrical field. As the gate-bias decreases (the quasi-Fermi level decreases, see Fig. 3c ), more holes are involved in the impact ionization process to generate more electron-hole pairs. Thus, there is a competing effect between the hole impact ionization and the direct photoexcitation. The former is more efficient than the latter when the material is converted to be more p -type. ( b ) Hole impact ionization process in the processed graphene photodetector. The rest mass energy of the hole in the high energy level h k is combined with the kinetic energy K h to create a lower-energy hole and electron-hole pairs as: h k + K h → h j + n × ( e + h ) where K h is the kinetic energy of holes induced by the external electric field. h k and h j indicate the higher-energy and the lower-energy level holes, respectively, ( e + h ) refer to electron-hole pairs and n is an integer. Thus, with an external electrical field, more electron-hole pairs can be generated through hole impact ionization. ( c ) The photoconductive gain spectra of Sample B and Sample C, respectively, at different photon excitation energies. The photoconductive gain rises as the photon energy increases, which can be attributed to the increase of the carrier MEG effect. With a higher photon energy excitation (532 nm), a photo-generated electron occupies a higher-energy level and generates multiple secondary electrons when scattering to the lower-energy levels in the conduction band through the MEG process, thus leading to a larger number of the captured electrons in the defect MGB. Full size image where K h is the kinetic energy of holes induced by the external electric field, h k and h j indicate the higher-energy and lower-energy level holes, respectively, ( e + h ) refer to electron-hole pairs, and n is an integer. As the gate-bias decreases (the quasi-Fermi level decreases), more holes are involved in the impact ionization process inducing more electron-hole pairs. Thus, there is a competing effect between the hole impact ionization and the direct photoexcitation for electron-hole pair generation. The former is more efficient than the latter when the material is converted to be more p -type. Figure 7c shows the photoconductive gain spectra of the Samples B and C with different average GQD sizes. For both devices, the photoconductive gain increases with the photon energy, arising from the increase of the carrier MEG efficiency. As the photo-excited electron occupies a higher-energy level in the conduction band under a shorter wavelength illumination (532 nm), it undergoes more exciton excitations through the impact ionization process when scattered into the lower-energy levels in the conduction band. This leads to an increase of the conduction-band electrons thus the captured electrons in the MGB as well, resulting in a higher photoconductive gain. In addition, Fig. 7c shows that the Sample B with a larger average GQD size (~20.5 nm) has a smaller photocurrent gain than the Sample C with a smaller average GQD size (~7.5 nm). As the size of the GQDs increases, the defect density decreases as evidenced in the Raman measurement results ( Fig. 3a ), resulting in a fewer number of photo-excited electrons captured by the MGB states. Theoretically, we can quite accurately calculate the photoconductive gain as a function of bias by the microscopic density matrix method [30] , but the microscopic analysis requires intensive derivations and accurate prediction of certain parameters, which are beyond the scope of this paper. Here we provide a simple macroscopic estimation on the photoconductive gain based on the population dynamic analysis. In our calculation, the source-drain bias and gate voltage are set as 20 mV and 0 mV, respectively. Here we assume the electron populations in the conduction band and the MGB are n 1 and n 2 , respectively. The recombination rate of electrons is R ~1 ps ( [45] ), the measured current is I , the capture rate of the MGB is α , the lifetime of the trapped electrons is τ 1 , the transition time is τ t , and the photogeneration rate is β . We assume the number of electrons per absorbed photon due to both electron and hole impact ionizations is χ . As the electron multiplication factor in perfect graphene sheet is estimated to be around four [30] , we reasonably assume that this factor in our device is not high neither. The hole impact ionization is not expected to be strong, as a zero gate voltage is applied resulting in a low hole density and a low drain-source voltage is applied. In this case, we assume the factor χ induced by both electron and hole impact ionizations is a small value <10. Under illumination, the variation of the number of the electrons in the conduction band originates from photogeneration, carrier multiplication (carrier impact ionization), recombination and relaxation to the MGB. The variation of the electrons on the MGB states results from excitation to the conduction band, relaxation from the conduction band, and recombination with holes in the valance band. Thus, we have From equations (2)–(4), the capture rate can be expressed as and the quantum efficiency η of the photo-excited and secondary-generated electrons captured by MGB is expressed as From equations (5) and (6), we obtain α is about 10 6 and η is about 10 −6 by applying appropriate values, where τ 1 is about 30 s obtained from Supplementary Fig. S3 and Supplementary Note 3 and τ t is about 250 ns achieved from Supplementary Fig. S4 . We can then calculate the photoconductive gain of the fabricated graphene photodetector by using [43] , which leads to a photoconductive gain of about 120. We could also calculate the photoconductive gain by G = N electrons / N photons where N electrons and N photons are the number of generated electrons that measured in the FET and the number of incident photons, respectively. We take the measured photocurrent of 6.961 nA and the visible irradiation of 5.57 nW on Sample C for calculation. A photoconductive gain of ~127 is obtained at a 20-mV source-drain bias and a zero gate voltage, in good agreement with that obtained from the above population dynamic analysis. We attribute the high and broadband photoresponse of our devices to the electron trapping in the defect MGB enhanced by the carrier impact ionization. We now discuss additional sets of reasons that address potential explanations of these findings. One is based on the ‘built-in-field’ scenario [6] , [7] , [14] , [46] . In this scenario, the slope of the I–V curve should keep a constant with and without illuminations, and the device should have a certain output photocurrent even when no bias is applied owing to the presence of the ‘built-in-field’ which separates the generated electron-hole pairs. In addition, the photoresponsivity should be at the level of several mAW −1 . These are in contrast to our observations. Another possible reason proposed in the literature is relied on the photo-thermoelectric effect [8] , [9] , [47] . This effect only occurs in asymmetric situations, either with asymmetric materials such as graphene p–n junctions or with asymmetric illuminations. In our case, the channel material is built by just a single layer graphene sheet (no junction exists) and the illumination is uniform. Therefore, none of the above explanations proposed in the literature can explain the observed high photoresponsivity. Our device covers a broad wavelength range, including the mid-infrared. The mid-infrared detector has wide applications ranging from medicine [48] , remote sensing [49] , environment monitoring [50] , to telecommunications [51] . The traditional mid-infrared HgCdTe and quantum well infrared photodetector photodetectors require complicated fabrication and growth of single-crystalline alloys using expensive molecular beam epitaxy or metalorganic chemical vapour deposition, thus the fabrication process is complex and has a high cost. The proposed graphene photodetector has a much lower cost and a lower operation voltage, and is compatible with the complementary metal-oxide-semiconductor technology. Despite the reported high photoresponsivity of our graphene photodetector over a broadband range, it needs to be mentioned that one drawback of the current device is that the operation speed is not high, which is mainly limited by the relatively long trapped electron lifetime in the defect states, caused by the present chemical fabrication/etching method introducing extremely complex deep surface and edge defects. The lifetime of the trapped electrons in the MGB is influenced by many factors, for example, defect types, trap-state density and defect trap depths. It has been demonstrated that by varying the types and the densities of defects one can significantly reduce the electron trap lifetime in various material systems [52] , [53] , [54] , [55] from tens of seconds down to a few milliseconds or even shorter. Thus we reasonably believe that the trapped electron lifetime in graphene can also be decreased by engineering the defect types and defect densities, for example, by achieving mechanically fabricated quantum dot edge defects with electron-beam lithography [16] or well-defined extended defects [22] using nickel supporting layer, or atomic-level nanoribbons with edge defects by a surface-assisted coupling method [32] . Certainly, by decreasing the lifetime of the trapped electrons, the photoresponsivity of the photodetector is sacrificed. This, however, can be compensated by increasing the low carrier mobility (caused by the VRH effect and the high defect scattering) in our highly disordered GQD array devices. This can be achieved by using more accurate fabrication techniques, for example, electron-beam lithography, helium ion lithography [56] , scanning tunnelling microscope lithography [57] and focused ions beam [58] to reduce the disorders and defect density, and by exploring other nanostructures such as nanoribbons and nanomeshs (without relying on the VRH effect), which are now under investigations. Therefore, we could conduct further band structure engineering of graphene to improve the operation speed as well as the temperature performance while still maintaining a high photoresponsivity of the proposed photodetector. In summary, we have demonstrated a new type of broadband pure monolayer graphene-based photodetector through band structure engineering. The demonstrated pure graphene photodetector shows a high photoresponsivity, which are about two–three orders of magnitude higher than those in the former reports. Compared with other band structure engineering approaches, the proposed fabrication method is simpler and a larger scale of device can be easily fabricated. Further device performance improvement can also be achieved through defect engineering and nanostructure engineering. The proposed scheme opens up exciting opportunities for band structure engineering of graphene for future graphene-based optoelectronic applications. Device fabrication We fabricated pure graphene photodetectors in a FET structure (inset, Fig. 3a ) for characterizations. First, a monolayer graphene was fabricated by using the micromechanical exfoliation technique on a 285-nm SiO 2 /Si substrate where the Si substrate is highly doped. Two electrode terminals (Ti/Au: 20 nm/80 nm), that is, the source and the drain terminals, were then formed by standard photolithography and lift-off techniques on top of the graphene. To clean the photoresist, Ar/H 2 annealing was applied at 400 degree for 2 h. Then, the gate terminal was fabricated on the bottom of the Si substrate. After that, a thin Ti sacrificial layer with different thicknesses was deposited by e-beam evaporation. Finally, the GQD array structures were formed by removing the Ti sacrificial layer using hydrofluoride, hydrodioxide (H 2 O 2 ) and deionized water with a volume ratio of 1:1:200 (the etching rate was around 20 nm min −1 ). The thicker the deposited Ti layer, the smaller the average size of the GQDs after etching. Thus the Ti sacrificial layer with various thicknesses can be deposited to control the average size of the GQDs. Device characterization Raman spectra measurements were used to characterize the density of defects of the fabricated devices ( Fig. 3a ). The Raman spectra were excited at 532 nm with an incident power <1 mW (laser spot diameter of 500 nm). For the pristine graphene sample (Sample A), the G-band and the 2D band are at 1,578 cm −1 and 2,666 cm −1 , respectively. For the processed graphene samples B and C, three defect-related Raman peaks are excited, namely D, D′ and D+D′ located around 1,338 cm −1 , 1,620 cm −1 and 2,934 cm −1 , respectively. The D and D′ peaks originate from double-resonance processes at the K point in the presence of defects, involving, respectively, intervalley (D) and intravally (D′) phonons [37] . A higher number of defects were observed in Sample C than in Sample B due to the higher Raman I D / I G ratio. As shown in Fig. 3b , after defects are introduced, the on-state electric conductance decreases to 0.14G 0 . Carrier transport in the device We measured the electrical properties of the devices at different temperatures ( Fig. 4a–c ). It is observed that the I – V characteristics of the processed graphene is linear at 294 K for V D changes from −1 V to 1 V, while it become remarkably nonlinear and highly symmetric, and the conductance reduces at low biases, at 12 K. These phenomena indicate the Coulomb blockade effect exists as carriers transport in the processed graphene sample. It is noted that the Schottky barrier formed between the contact and the graphene layer could also generate a decreased conductance at a lower bias, but this effect is excluded because it would also introduce a nonlinear effect at room temperature and an asymmetric behaviour at low temperatures [41] , which are not observed in our measurements. This means the observed phenomena comes from the graphene FET channel. Photoresponse measurement The photoresponsivity measurement was performed in a digital deep level transient spectroscopy (BIORAD) system with a compressor (CTI-CRYOGENICS, 8200). Three light sources (visible: 532 nm semiconductor laser; near-infrared: 1470 nm fibre laser; mid-infrared: tunable quantum cascade laser from 9.75 to 10.48 μm) were used to illuminate the whole device. The electrical characteristics were collected by a semiconductor device analyser (Agilent, B1500A). How to cite this article: Zhang, Y. et al . Broadband high photoresponse from pure monolayer graphene photodetector. Nat. Commun. 4:1811 doi: 10.1038/ncomms2830 (2013).